Observations of ubiquitous compressive waves in the Sun’s chromosphere The details of the mechanism(s) responsible for the observed heating and dynamics of the solar atmosphere still remain a mystery. Magnetohydrodynamic waves are thought to have a vital role in this process. Although it has been shown that incompressible waves are ubiquitous in off-limb solar atmospheric observations, their energy cannot be readily dissipated. Here we provide, for the first time, on-disk observation and identification of concurrent magnetohydrodynamic wave modes, both compressible and incompressible, in the solar chromosphere. The observed ubiquity and estimated energy flux associated with the detected magnetohydrodynamic waves suggest the chromosphere is a vast reservoir of wave energy with the potential to meet chromospheric and coronal heating requirements. We are also able to propose an upper bound on the flux of the observed wave energy that is able to reach the corona based on observational constraints, which has important implications for the suggested mechanism(s) for quiescent coronal heating. The quiet chromosphere is a highly dynamic region of the Sun’s atmosphere. It consists of many small-scale, short-lived, magnetic flux tubes (MFTs) composed of relatively cool (10 4 K) plasma [1] . The quiet chromosphere may be divided into two magnetically distinct regions [2] . One is the network, which generally consists of open magnetic fields outlined by plasma jets, that is, spicules and mottles, which protrude into the hot (10 6 K) corona. The other region is the inter-network that is populated by fibrils that outline magnetic fields, joining regions of opposite polarity and that are hence closed within the chromosphere [1] , [3] , [4] . The possible importance of chromospheric dynamics on the upper atmosphere has recently been highlighted by joint Hinode and Solar Dynamic Observatory [5] measurements and ground-based observations by the Swedish Solar Telescope [6] , showing a direct correspondence between chromospheric structures and plasma that is heated to coronal temperatures. Magnetohydrodynamic (MHD) waves have long been a suggested mechanism for distributing magneto-convective energy, generated below the solar surface, to the upper layers of the Sun's atmosphere [7] , [8] . Incompressible MHD wave modes, characterized by the transverse motions of the magnetic field lines, have been observed to be ubiquitous throughout the solar chromosphere [9] , [10] , [11] and corona [12] , [13] , [14] . However, incompressible wave energy is notoriously difficult to dissipate under solar atmospheric conditions [15] , requiring very large Alfvén speed gradients occurring over short (sub-resolution) spatial scales to achieve the necessary rate of plasma heating. In contrast, compressible MHD waves are readily dissipated by, for example, compressive viscosity and thermal conduction [15] . Active region fast compressible MHD waves have recently been identified at both photospheric and coronal heights [16] , [17] , [18] . There has been some tentative evidence for their existence in the quiet chromosphere [19] , but now we establish their ubiquity in this paper, making them a possible candidate for plasma heating in the quiescent corona. We demonstrate here the presence of concurrent, ubiquitous, fast compressive MHD waves and incompressible MHD waves in the on-disk solar chromosphere. Measurements of the wave properties (that is, period, amplitude and phase speed) for both compressible and incompressible modes are provided. Further, we derive estimates for the flux of wave energy by combining advanced MHD wave theory and the observed wave properties. These estimates hint that the observed waves could have a crucial role in the transport of magneto-convective energy in the solar atmosphere. Chromospheric fine structure High spatial (150 km) and temporal resolution (8 s) observations with the Rapid Oscillations in the Solar Atmosphere (ROSA) imager [20] have allowed us to resolve the chromospheric structures and measure fine-scale wave-like motions therein. The data were obtained close to disk centre with a narrowband 0.25 Å Hα core (6562.8 Å) filter on the 29 September 2010 (see Methods for further information on the processing of the observational data). The field of view covers a 34 Mm × 34 Mm region of the typical quiet Sun ( Fig. 1 , Supplementary Fig. S1 ). The Hα core images are known to show the mid- to upper chromosphere where the magnetic pressure dominates the gas pressure [3] , [21] . The images ( Supplementary Movie 1 ) show that the on-disk chromosphere is dominated by hundreds of bright and dark fine structures, all displaying highly dynamic behaviour. The elongated structures are the fibrils and shorter structures are the mottles. Recent advances in the modelling of Hα line formation suggest the dark structures are regions of enhanced density that closely follow the magnetic field structure [22] . The nature of the bright fine structures is less clear, although they are suspected to be similar to the dark features except for differences in their gas pressure [23] . In Fig. 1 we show the measured widths of over 300 bright and dark structures, and the results demonstrate the geometric similarity between these structures. 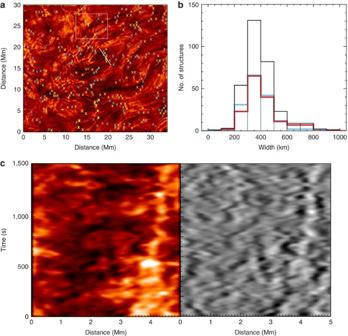Figure 1: Observed chromospheric structures and their transverse motions. (a) The ROSA Hα field of view att=0 s. Blue and yellow crosses mark positions of identified dark and bright chromospheric MFTs, respectively. The boxed region is where the chromospheric structures inFig. 4are observed. (b) Histogram of measured MFT widths. Blue and red lines correspond to the dark and bright MFTs, respectively. The black line is the combined result with a mean width of 360±120 km. (c) Time-distance plot (left) and median filtered version (right) taken across a group of chromospheric structures. The cross-cut used is shown in (a). The given distance starts from the bottom of the cross-cut and the time is in seconds from the beginning of the data set. The dark and bright linear tracks are the transverse motions of the structures. Figure 1: Observed chromospheric structures and their transverse motions. ( a ) The ROSA Hα field of view at t =0 s. Blue and yellow crosses mark positions of identified dark and bright chromospheric MFTs, respectively. The boxed region is where the chromospheric structures in Fig. 4 are observed. ( b ) Histogram of measured MFT widths. Blue and red lines correspond to the dark and bright MFTs, respectively. The black line is the combined result with a mean width of 360±120 km. ( c ) Time-distance plot (left) and median filtered version (right) taken across a group of chromospheric structures. The cross-cut used is shown in ( a ). The given distance starts from the bottom of the cross-cut and the time is in seconds from the beginning of the data set. The dark and bright linear tracks are the transverse motions of the structures. Full size image The observed structures can be considered as discrete over-dense MFTs outlining the magnetic field, embedded in a less dense ambient plasma. They are short-lived (1–5 min) but fortunately survive long enough to allow measurements of important wave parameters, for example, velocity amplitude and propagation speed. The observations show that similar structures re-occur in the same regions either continuously or even tens of minutes after previous structures have faded from the field of view ( Supplementary Movies 1 and 2 ), suggesting that the lifetime of the background magnetic field is much longer than the plasma flows that generate the visible structuring. Waves may be present in the atmosphere even when the magnetic field is not outlined by an intensity enhancement; however, they are far more difficult to identify directly. These intensity enhancements suggest a greater plasma density along the waveguide relative to the surrounding atmosphere, which has important physical effects on the properties of the wave. Mathematically, it is well-known that plasma structuring in solar waveguides, even if modelled as relatively simple over-dense cylindrical MFTs, can produce an infinite set of orthogonal eigenmodes [24] , [25] . This is in stark contrast to only three possible modes of a homogeneous magnetized plasma (Alfvén, fast and slow magnetosonic modes). Although the full MHD spectrum of permitted wave modes in realistic inhomogeneous solar MFTs is rich and complex, in practice, due to limits in spatial resolution, most of the wave power observed so far has been confined to the low order azimuthal wave number modes, that is, torsional Alfvén, sausage and kink. Higher order fluting modes predicted by theory, to our knowledge, have yet to be detected in solar data. It has, however, been suggested by numerical simulations that different MHD wave modes should occur simultaneously in chromospheric MFTs [26] . In this current work, we identify such concurrent wave modes. Incompressible transverse waves To analyse the waves, a cross-cut is placed perpendicular to a chromospheric structure’s axis and time-distance plots are constructed (for example, Fig. 1 , Supplementary Figs S2 and S3 ). We find that the chromospheric structures support two concurrent orthogonal MHD wave modes. The first type is the transverse motion of the structure’s axis ( Fig. 2 ), which is ubiquitous and even visible by eye ( Supplementary Movies 1–4 ). In terms of the over-dense magnetic waveguide model, we interpret these motions as the highly incompressible MHD fast kink wave [24] , [25] . The transverse displacements appear predominantly as linear, diagonal tracks in the time-distance plots, although occasionally leaving sinusoidal tracks (see Methods for further details). The properties of over a hundred representative transverse motions were measured and they reveal that the typical displacement amplitudes are 315±130 km with velocity amplitudes of 5–15 km s −1 ( Fig. 3 ). For isolated chromospheric structures (for example, those in Fig. 4 and Supplementary Fig. S2 ) a Gaussian can be reliably fitted to the cross-sectional flux profile to obtain the transverse displacement and velocity amplitudes, and the period (see Methods for further details). A linear fit to the diagonal tracks is undertaken when a Gaussian fit cannot be performed. The number of structures to which a Gaussian fit can be applied is 47; the remainder of the fits are linear. Using cross-correlation, the propagation speeds can also be measured and values in the range 40–130 km s −1 are obtained ( Supplementary Table S1 ). We note that the amplitude and period of the waves observed here are similar to those reported in limb observations of spicules [10] . The amplitudes of the transverse motions are of the order of, or greater than, the waveguide width (360 km), implying that they are fast kink wave modes in the nonlinear regime. 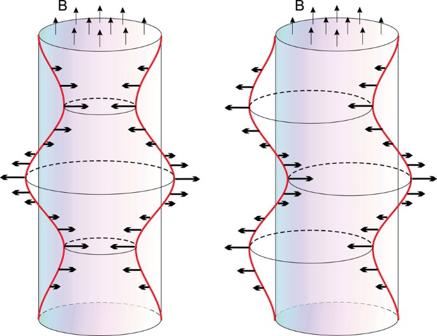Figure 2: Schematic diagrams of MHD waves in an MFT. The MHD wave modes supported by the chromospheric fine structure can be modelled as a cylindrical magnetic waveguide. The fast MHD sausage wave (left) is characterized by a periodic contraction and expansion of the MFTs cross-section symmetric about the central axis, stretching and squeezing the magnetic field. This, in turn, induces a decrease and increase in the plasma pressure inside the MFT that changes the intensity of the observed MFT in the Hα bandpass. The fast MHD kink wave (right) displaces the central axis of the MFT. The red lines show the perturbed waveguide and thick arrows show the velocity amplitudes. The thin arrows labelled B show the direction of the background magnetic field. Figure 2: Schematic diagrams of MHD waves in an MFT. The MHD wave modes supported by the chromospheric fine structure can be modelled as a cylindrical magnetic waveguide. The fast MHD sausage wave (left) is characterized by a periodic contraction and expansion of the MFTs cross-section symmetric about the central axis, stretching and squeezing the magnetic field. This, in turn, induces a decrease and increase in the plasma pressure inside the MFT that changes the intensity of the observed MFT in the Hα bandpass. The fast MHD kink wave (right) displaces the central axis of the MFT. The red lines show the perturbed waveguide and thick arrows show the velocity amplitudes. The thin arrows labelled B show the direction of the background magnetic field. 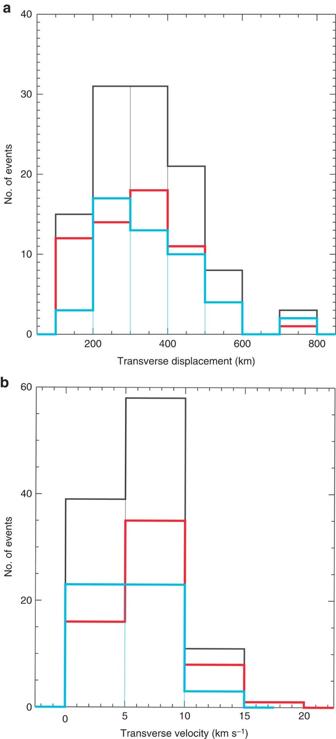Figure 3: Measured properties of transverse displacements and velocity amplitudes for the fast MHD kink mode. (a) The distribution of transverse displacements of 103 chromospheric structures measured using linear fits to the observed tracks. The blue and red lines correspond to dark and bright structures, respectively. The black line shows the combined results with a mean displacement of 315 km and s.d. of 130 km. (b) Velocity amplitudes for both bright and dark chromospheric structures. The transverse velocity has a mean value of 6.4 km s−1with a s.d. of 2.8 km s−1. The dark and bright structures show a similar distribution. Full size image Figure 3: Measured properties of transverse displacements and velocity amplitudes for the fast MHD kink mode. ( a ) The distribution of transverse displacements of 103 chromospheric structures measured using linear fits to the observed tracks. The blue and red lines correspond to dark and bright structures, respectively. The black line shows the combined results with a mean displacement of 315 km and s.d. of 130 km. ( b ) Velocity amplitudes for both bright and dark chromospheric structures. The transverse velocity has a mean value of 6.4 km s −1 with a s.d. of 2.8 km s −1 . The dark and bright structures show a similar distribution. 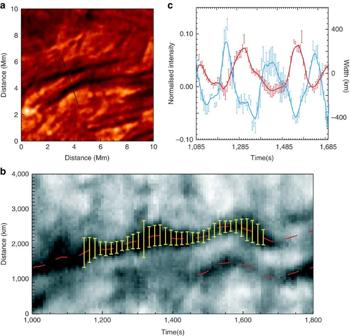Figure 4: Concurrent wave modes in chromospheric structures. (a) Typical ROSA Hα example of a pair of relatively large dark flux tubes att=1,536 s measured from the beginning of the data series. (b) Time-distance plot revealing the dynamic motion. The position of the cross-cut is shown in (a), with the given distance starting at the top of the cross-cut. Times are given in seconds from the start of the data set. The results from a Gaussian fitting are over-plotted and show the nonlinear fast MHD kink wave (red line shows the central axis of the structure) and the fast MHD sausage mode (yellow bars show the measured width of structure). The transverse motion has a period of 232±8 s and we detect multi-directional propagating transversal wave trains in the MFT travelling with speeds of 71±22 km s−1upwards and 87±26 km s−1downwards (for further details, seeSupplementary Fig. S6). The typical velocity amplitudes are 5 km s−1. The fast MHD sausage mode has a period of 197±8 s, a phase speed of 67±15 km s−1and apparent velocity amplitudes of 1–2 km s−1. (c) Comparison of MFTs intensity (blue) and width (red) perturbations from the Gaussian fitting. The data points have been fitted with a smoothed 3-point box-car function. The observed out-of-phase behaviour is typical of fast MHD sausage waves. The error bars plotted are the one-sigma errors on each data point calculated from the Gaussian fitting. Full size image Figure 4: Concurrent wave modes in chromospheric structures. ( a ) Typical ROSA Hα example of a pair of relatively large dark flux tubes at t =1,536 s measured from the beginning of the data series. ( b ) Time-distance plot revealing the dynamic motion. The position of the cross-cut is shown in (a), with the given distance starting at the top of the cross-cut. Times are given in seconds from the start of the data set. The results from a Gaussian fitting are over-plotted and show the nonlinear fast MHD kink wave (red line shows the central axis of the structure) and the fast MHD sausage mode (yellow bars show the measured width of structure). The transverse motion has a period of 232±8 s and we detect multi-directional propagating transversal wave trains in the MFT travelling with speeds of 71±22 km s −1 upwards and 87±26 km s −1 downwards (for further details, see Supplementary Fig. S6 ). The typical velocity amplitudes are 5 km s −1 . The fast MHD sausage mode has a period of 197±8 s, a phase speed of 67±15 km s −1 and apparent velocity amplitudes of 1–2 km s −1 . ( c ) Comparison of MFTs intensity (blue) and width (red) perturbations from the Gaussian fitting. The data points have been fitted with a smoothed 3-point box-car function. The observed out-of-phase behaviour is typical of fast MHD sausage waves. The error bars plotted are the one-sigma errors on each data point calculated from the Gaussian fitting. Full size image Fast compressible waves The second type of dynamic behaviour in chromospheric structures ( Fig. 2 ), concurrent with the transverse displacement ( Figs 4 and 5 , Supplementary Figs S2 and S4 ), is a periodic increase and decrease of the structures’ intensity. In conjunction, there is an anticorrelated contraction and expansion of the structures’ visible cross-section. Both the intensity and width perturbations are obtained from the Gaussian fits. This perturbation is found to propagate along chromospheric structures with speeds much greater than the sound speed and is comparable to the local Alfvén speed (see Methods for further details). We interpret the observed periodic changes in intensity from MHD wave theory [24] , [25] as being consistent with the compressive properties of the fast MHD sausage mode. The visible lifetime of the chromospheric structures are also comparable to the fast sausage and kink modes’ period, which means that observing multiple wave cycles is rather difficult. However, the fast propagating intensity disturbances can also be identified in time-distance diagrams that are constructed when a cross-cut is placed parallel to a structure’s axis (see Fig. 5 , Supplementary Figs S4, S5 and S6 ). These events are seen to occur continuously all over the field of view ( Supplementary Movies 3 and 4 ). A table of measured phase speeds and periods is provided in Supplementary Table S2 . 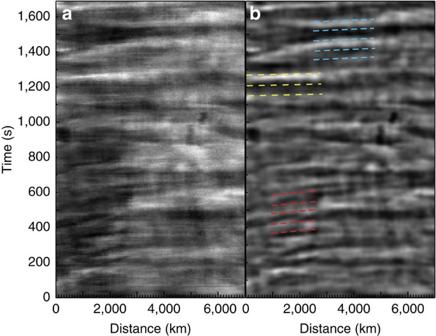Figure 5: Fast propagating intensity perturbations (a) A typical time-distance diagram obtained by placing a cross-cut parallel to a chromospheric structure. This particular cross-cut is perpendicular to the cross-cut shown inFig. 1a. (b) The same time-distance plot is shown as in (a) but it has been subject to a median filter. The result reveals periodic variations in intensity that propagate along the cross-cut, hence the chromospheric structure. Measuring the gradients of the tracks created by the intensity perturbations across the time-distance plots provides propagation velocities. The coloured, dashed lines highlight three examples of these periodic variations. The measured propagation velocities are 78±9 km s−1(red), 270±135 km s−1(yellow) and 135±17 km s−1(blue). The amplitude of the perturbation in intensity is ≤10% of the background value, similar to that found from the Gaussian fitting (Fig. 4). Figure 5: Fast propagating intensity perturbations ( a ) A typical time-distance diagram obtained by placing a cross-cut parallel to a chromospheric structure. This particular cross-cut is perpendicular to the cross-cut shown in Fig. 1a . ( b ) The same time-distance plot is shown as in (a) but it has been subject to a median filter. The result reveals periodic variations in intensity that propagate along the cross-cut, hence the chromospheric structure. Measuring the gradients of the tracks created by the intensity perturbations across the time-distance plots provides propagation velocities. The coloured, dashed lines highlight three examples of these periodic variations. The measured propagation velocities are 78±9 km s −1 (red), 270±135 km s −1 (yellow) and 135±17 km s −1 (blue). The amplitude of the perturbation in intensity is ≤10% of the background value, similar to that found from the Gaussian fitting ( Fig. 4 ). Full size image Interestingly, the sausage mode has distinct regimes that define whether the majority of wave energy can be trapped in the vicinity of a density enhancement along the magnetic field or it leaks away [24] , [25] , [27] . To investigate whether the observed fast MHD sausage modes are mostly trapped or leaky we have to estimate if the product of wave number ( k ) and waveguide half-width ( a ) is a sufficiently small parameter. For the observed chromospheric structures the sausage mode would have to have ka >0.2 to be trapped but we observe, for example, in Fig. 4 , that ka ∼ 0.08±0.03 (see Supplementary Discussion for further details). Therefore, the observed sausage modes appear to be in the leaky regime, further enhancing their already dissipative nature. It is important to note that leaky sausage modes, with no damping due to physical effects such as compressive viscosity or radiation, would still radiate energy away from the waveguide with decay times on the order of the period. Now, let us estimate the energy flux for the observed MHD waves using the waveguide model. The polarization relations for a particular wave mode allow us to determine the perturbations of all the relevant physical quantities, if we know the perturbation of one [24] , [25] . This way we obtain an estimate for the amplitude of the perturbations we cannot measure directly otherwise, for example, the magnetic field fluctuations (see Supplementary Methods for further details). The polarization relations need to be supplemented with typical values of chromospheric plasma parameters (for example, density [1] , [22] , ρ =3 × 10 −10 kg m −3 , temperature [22] , [23] , T =10,000 K and magnetic field strength [28] , B =10 −3 T) and the amplitudes and phase speeds measured here. The time-averaged wave energy flux in the chromospheric plasma is composed of two dominant components, the kinetic and the magnetic energy flux, < E > =c ph [ ρ v 2 + b 2 / μ 0 ]/4, where v and b are the amplitudes of the velocity and magnetic perturbations, respectively, c ph is the phase speed and μ 0 is the magnetic permeability of free space. The thermal energy contributions from each mode are found to be negligible due to the magnetic pressure being at least an order of magnitude greater than the gas pressure in the chromosphere. The estimated energy flux of the incompressible fast kink mode is 〈 E k 〉=4,300±2,700 W m −2 , which is comparable to that estimated in off-limb spicules [9] . The estimated wave energy flux for the compressible fast MHD sausage mode is 〈 E s 〉 =11,700±3,800 W m −2 per chromospheric structure for apparent radial velocity amplitudes of v ∼ 1–2 km s −1 . The details of the wave energy calculation applicable to the observed inhomogeneous structured plasma are given in the Supplementary Methods , Supplementary Figs S7 and S8 and Supplementary Table S3 . A further comment on the wave energy flux is required. The over-dense cylindrical waveguide supports different MHD wave modes, where some, but not all, of the energy of trapped modes is concentrated near the waveguide. Consequently, the consideration of collections of over-dense waveguides occupying the chromosphere results in a much more complex calculation of the total energy flux. The derived value does not take into account the following: the wave energy of leaky modes is not confined within the flux tube, with a comparable amount of perturbation energy outside the tube. This means calculation of the internal wave energy flux only, leads to an underestimate; only a linear approach for the wave energy flux is given. The transverse motions are generally observed to be strongly nonlinear, so we are underestimating the wave energy flux by ignoring these nonlinear terms; the true nature of the chromospheric fine structure is difficult to determine at present. The homogeneous cylindrical model is a simplifying assumption and does not account for the true geometry of the structure and/or any radial structuring of the plasma. All the above factors could influence the energy estimates. Calculating the total wave energy in a plasma such as the chromosphere is complex and will require further observations and full three-dimensional MHD numerical simulations before improved values for wave energy flux can be obtained. Knowing the eventual fate of the wave energy observed in the chromosphere is vital in assessing which (if any) wave-based heating models are likely candidates for explaining the long-standing solar atmospheric heating puzzle [29] , [30] , [31] , [32] , [33] , [34] , [35] . Using the measured properties of the chromospheric structures, we estimate (see Supplementary Discussion for further details) that a maximum of 4–5% of the chromospheric volume is connected by MFTs that protrude into the corona. This estimate of connectivity between the chromosphere and corona is subject to observational constraints but the given value may not change significantly with improved spatial resolution. The estimated connectivity suggests that the total energy flux across the solar surface able to reach the corona from the chromosphere is ∼ 170±110 W m −2 for the incompressible transverse motions and ∼ 460±150 W m −2 for compressive motions. The estimate for chromospheric transverse wave energy able to reach the lower corona agrees with the energy estimates in the same period range (100–500 s) from off-limb Solar Dynamic Observatory quiet Sun observations [14] , which could suggest that these waves remain relatively undamped on their journey. This can be explained by the known difficulty of dissipating these incompressible waves [15] . As it is expected that the majority of field lines observed here remain closed (that is, the fibrilar structure), this suggests that the observed chromospheric wave energy remains largely in the chromospheric volume to be dissipated in a different manner [33] , [34] , [35] . On the other hand, the eventual fate of the chromospheric fast compressive waves is still unclear. However, our results imply that the waves could have a significant role in meeting chromospheric ( ∼ 10 kW m −2 , [36] ) and quiet coronal heating requirements (100–200 W m −2 , [36] , [37] ). Further work is needed to: provide more representative statistics on typical perturbation amplitudes of the fast compressive waves, which will lead to improved estimates for the energy flux of the waves; search for coronal counterparts of the sausage MHD waves in the corona; and assess how the leaky nature of the waves affects the wave energy transmission to and dissipation in the lower corona. The observations presented here demonstrate that the on-disk quiet chromosphere, which is dominated by fibrilar structure, supports ubiquitous incompressible transverse waves. The properties of the transverse waves observed agree with those reported to exist in limb spicules [10] , which are magnetic waveguides that penetrate into the low corona. This points towards a close connection between the disk and limb structures even if their magnetic topology (that is, open or closed magnetic fields) is potentially different. In addition, the observation and identification of ubiquitous, fast propagating, compressible MHD waves demonstrates that the chromosphere is replete with MHD wave energy. The ubiquity of both the incompressible and compressible waves, in conjunction with our initial estimates of wave energy, gives further credence to models of a predominantly wave-based quiescent atmospheric heating mechanism. Observational set-up and data processing The data was obtained at 15:41–16:51 UT on 29 September 2010 with the Dunn Solar Telescope at Sacremento Peak, USA. The six-camera system ROSA was employed. ROSA observed a 69″.3 by 69″.3 region of the quiet solar atmosphere in Hydrogen-α (6562.8 Å). The Hα filter is centred at the line core and a narrow bandpass (0.25 Å) is employed to ensure that photospheric contributions from the line wings are minimized (for details on Hα line formation see, for example, [3] , [21] , [22] ). During the observations, high-order adaptive optics [38] was used to correct for wave front deformation in real time. The seeing conditions were good. The data suffers from a period of poor seeing during the middle of the run lasting 300 s. The frames in this period of bad seeing are not used for analysis. The Hα data was sampled at 2.075 frames s −1 and image quality improved through speckle reconstruction [39] utilizing a 16−1 ratio, giving a final cadence of 7.68 s. To ensure accurate coalignment between frames, the narrowband time series were Fourier coregistered and de-stretched using vectors derived from longer-lived broadband stuctures [40] . Gaussian fitting of chromospheric structures We discuss here the procedure used to observe the periodic phenomena in the chromospheric magnetic structures. First, we place cross-cuts perpendicular to the structure’s central axis and obtain time-distance diagrams as shown in Figs 1 and 4 and Supplementary Fig. S2 . In each time slice, t , of the time-distance plot we fit a Gaussian profile to the cross-sectional flux profile, F ( x , t ), of the chromospheric magnetic structure, where the Gaussian fit is given by Here, f 0 ( t ) is the peak flux, f 1 ( t ) is the central position of the Gaussian, f 2 ( t ) is the Gaussian width and f 3 ( t ) is the background flux. The obtained fit parameters relate to the periodic motions: f 0 ( t ) gives intensity (or flux) perturbation; f 1 ( t ) gives the displacement of the structure’s central axis, that is, the transverse waves; f 2 ( t ) gives the full-width half-maximum (FWHM), 2 f 2 (2 ln 2) 1/2 , of the structure’s visible cross-section. Before measuring the properties (for example, period, velocity amplitude, so on) of each series f 0 , f 1… , each time series is de-trend by fitting a cubic function and subtracting the trend. The periods of the wave motion are obtained by using wavelet analysis. Examples of structures demonstrating periodic phenomenon derived from the Gaussian fits are shown in Fig. 4 and Supplementary Fig. S1 . The Gaussian fit is applied only to isolated chromospheric flux tubes to avoid the influence of the chromospheric structures crossing each other, which would lead to changes in both intensity and width. All errors provided with respect to the results obtained from the Gaussian fitting (that is, those in Fig. 4 , Supplementary Table S1 ) are one s.d. Measuring transverse amplitudes Here we discuss how the transverse amplitudes are obtained for the histograms in Fig. 3 . In the time-distance diagrams a large number of diagonal tracks ( Fig. 1 , Supplementary Fig. S3 ), with varying gradients, and a smaller number of sinusoidal tracks (for example, Fig. 4 , Supplementary Fig. S2 ) can be identified. These are the transverse motions of the chromospheric structures. The transverse amplitudes are obtained by measuring the length of the bright or dark diagonal tracks and the time-averaged velocity amplitudes are the gradients of the tracks. The Gaussian fit is not used here for determining the centre of the chromospheric structure. The spatial position of the centre of the chromospheric structures can be measured to the nearest pixel by locating the maximum/minimum value of intensity, which provides an error of 50 km on position. The time coordinate for each position of the chromospheric structure can only be known to within a range of 7.68 s, hence the error is dt ∼ ±3.84 s. For the measured values of displacement amplitude given in Fig. 3 the median value of the error is ∼ 13% of the given value. The velocity amplitude has a median error of 22% of the given value, which equates to 1.3 km s −1 and a s.d. on the error of 1.1 km s −1 . Calculating the velocity amplitude from the straight line fits only provides the time-averaged value of the amplitude. If a number of oscillatory cycles can be observed, then the following relation is used to find the maximum velocity amplitude, Here ξ r is the transverse displacement (given by f 1 in the Gaussian fit), v r is the radial velocity perturbation and P is the period of the oscillation. Only a small percentage of the observed oscillations show full cycles, that is, sinusoidal motions in the time-distance plots. The reason why we do not see full cycles is due to the relatively short lifetimes (1–5 min) of the chromospheric magnetic structures compared with a typical period of the fast kink waves (3 min). A similar behaviour is observed for limb spicules [9] , [10] . Amplitudes of the fast MHD sausage mode Here we describe how we estimate the velocity component of the fast MHD sausage mode from the changes in the FWHM as established by the Gaussian fitting. We assume that the compressive motion is a symmetric perturbation about the central axis of the waveguide. The FWHM is a measure of the chromospheric structure’s visible diameter. We make the assumption that the displacement in the radial direction occurs at the same rate as the change in the value of the FWHM. The radial velocity amplitude is given by equation (2) and we assume ξ r FWHM /2. Equation (2) can only be used when a number of cycles of the fast sausage mode are observed. The value for v r is the value of maximum amplitude. The time-averaged value is given by . We note that the assumption regarding the relationship between FWHM and the radial velocity may not hold true if the change in the visible cross-section does not accurately represent the physical change in cross-section. Detailed simulations of waves in plasmas and their influence on Hα line formation may be needed to resolve such issues. Fast propagating intensity disturbances The spatial resolution of ROSA ( ∼ 150 km) is close to the widths of the chromospheric flux tubes ( ∼ 350 km), making the joint detection of periodic changes in intensity and the width of flux tubes difficult to observe. However, it is possible to identify the fast compressive wave mode through identification of periodic, propagating intensity disturbances ( Fig. 5 , Supplementary Figs S4, S6 ). The intensity variations seen in the filtered data is ≤10% of the median intensity of the unfiltered intensity. This variation in intensity is in agreement with the values obtained from the Gaussian fits (compare Fig. 4 and Supplementary Fig. S2 ). From these filtered time-distance plots we are able to measure propagation speeds and periods of the observed periodic disturbances (see Supplementary Table S2 ). We identify 10 regions in which the properties of the fast propagating features can be measured ( Supplementary Fig. S6 ). We are confident the observed perturbations are due to the fast sausage modes as the periodic features have a large spatial coherence (>1000, km; see Supplementary Movies 3 and 4 ). This behaviour is somewhat expected due to the leaky nature of the oscillations (see Supplementary Discussion for further details). In contrast, the observed kink motions have a small spatial coherence (see Fig. 1 ), with neighbouring flux tubes showing little or no coherence. Measuring phase speeds To measure the phase speed for the observed waves in chromospheric structures, we have to be able to track the periodic variation in displacement and intensity, at different positions along the structure. We place cross-cuts at different positions along the structure’s central axis and fit a Gaussian to the observed sinusoidal variations. The time lag between the perturbed quantities obtained from the Gaussian fit in the different cross-cuts is obtained by using cross-correlation to calculate the shift between two signals. The phase speed is given as the average velocity determined from the time lags between different cross-cuts (see Supplementary Methods for further details) and the error is the s.d. The propagating nature of the waves is also seen by plotting the transverse displacement for different cross-cuts (as measured with the Gaussian fits). An example of this is shown in Supplementary Fig. S5 , where the propagation of the transverse wave shown in Fig. 4 can be seen. The distance between the displayed cross-cuts is ∼ 150 km. We note that it is possible that the phase speed varies as a function of distance along the structure due to density and magnetic field stratification; however, a combination of the technique used and the spatial and temporal resolution of the current observations does not allow us to determine this variation of phase speed. The phase speeds for the fast compressive disturbances are calculated differently. Once a periodic propagating disturbance is identified in time-distance plot (for example, Fig. 5 , Supplementary Fig. 4 ), the minimum or maximum valued pixel in time (depending on whether the maximum or minimum of the intensity perturbation is being measured) in each spatial slice is located. The gradient of a linear fit to the minimum/maximum values gives the phase speed. The errors on the spatial locations are 50 km and the time coordinates are 3.84 s. As the propagating disturbances are seen over relatively long distances for short periods of time, the largest source of error comes from the uncertainty in time. How to cite this article: Morton, R.J. et al . Observations of ubiquitous compressive waves in the Sun’s chromosphere. Nat. Commun. 3:1315 doi: 10.1038/ncomms2324 (2012).